Facile synthesis of pentacle gold–copper alloy nanocrystals and their plasmonic and catalytic properties The combination of gold and copper is a good way to pull down the cost of gold and ameliorate the instability of copper. Through shape control, the synergy of these two metals can be better exploited. Here, we report an aqueous phase route to the synthesis of pentacle gold–copper alloy nanocrystals with fivefold twinning, the size of which can be tuned in the range from 45 to 200 nm. The growth is found to start from a decahedral core, followed by protrusion of branches along twinning planes. Pentacle products display strong localized surface plasmon resonance peaks in the near-infrared region. Under irradiation by an 808-nm laser, 70-nm pentacle nanocrystals exhibit a notable photothermal effect to kill 4T1 murine breast tumours established on BALB/c mice. In addition, 70-nm pentacle nanocrystals show better catalytic activity than conventional citrate-coated 5-nm Au nanoparticles towards the reduction of p -nitrophenol to p -aminophenol by sodium borohydride. Through mixing two or more species, the scope of properties of metal nanocrystals can be significantly extended owing to various synergistic effects [1] , [2] , [3] , [4] , [5] , [6] , [7] , [8] , [9] , [10] . For example, forming hybrid, core-shell or alloy structures leads to affluent and interesting chemical and physical characteristics especially in catalysis and optics for both fundamental study and niche applications [11] , [12] , [13] , [14] , [15] , [16] , [17] , [18] , [19] . As a particular species of great service, gold nanocrystals exhibit unique and often tunable properties such as localized surface plasmon resonance (LSPR), biocompatibility, easy surface modification and catalytic effect towards many important oxidization reactions, which promote their comprehensive applications such as photothermal therapy, cancer diagnosis, imaging, drug delivery and pollution control [20] , [21] . As another coinage metal, copper share many well-defined shapes discovered for Au when forming nanocrystals [22] , [23] , [24] , [25] , [26] , [27] . Analogous to Au and other noble metals, Cu nanocrystals can display strong LSPR absorption in the spectral range of visible and near-infrared (NIR) [26] , [27] . However, the susceptibility of Cu upon exposure to air complicates the synthesis and applications of Cu nanocrystals. Therefore, the combination of Au and Cu will predictably pull down the high cost of Au and ameliorate the instability of Cu towards oxidization. There have been a few reports in literature on the synthesis of well-defined Au–Cu bimetallic nanocrystals [28] , [29] , [30] . Liu and Walker achieved the production of Au–Cu alloy nanocubes through a one-pot polyol strategy [28] . They found that the LSPR wavelength of nanocubes was highly dependent on size and composition. Chen et al . reported a protocol employing the diffusion of newly reduced active Cu atoms into pre-synthesized Au seeds to prepare intermetallic Au–Cu nanocrystals [29] . Distinct from solid-state diffusion, the solution phase, atomic-scale diffusion is homogeneous and generates uniform and monodisperse products. Apart from using chemical methods, Yin et al. [30] reported the preparation of mass-selected Au–Cu core-shell clusters containing several thousand atoms through a magnetron-sputtering gas phase method. By manipulating the condensation parameters, size, composition and structure of the bimetallic nanocrystals can be controlled. Despite these remarkable demonstrations, Au–Cu bimetallic nanocrystals that have been reported are limited in well-defined shape and are mostly enclosed by low-index facets including {111}, {100} and {110}. Since controlling the crystalline structure and exposed facets of metal nanocrystals have always provided a powerful means to modulate their properties, there is a unremitting drive to pursue diverse interesting shapes, for instance, nanocrystals with multiple branches. In general, highly branched nanocrystals enjoy higher surface-to-volume ratio and possibly rougher surfaces than their more isotropic counterparts, both of which can avail surface-sensitive applications such as LSPR and catalysis [31] , [32] , [33] . In addition, it has been pointed out that nanostructures with branched arms on the surface are often endowed with high-index feature [34] , [35] , [36] , [37] . High-index facets relate to a high density of atomic steps, kinks and edges with low coordination numbers, which can act as highly active sites for breaking chemical bonds [33] , [34] , [35] , [36] , [37] . Since limited success has been accomplished in the synthesis of bimetallic nanocrystals with multiple branches, it is of significant value to investigate the synergy between Au, Cu and branched shape, which can probably uphold the application of Au–Cu bimetallic nanocrystals. Herein we present a facile approach to size-controlled synthesis of pentacle Au–Cu alloy nanocrystals with fivefold twinning in aqueous solution. By adjusting the amount of capping agent, we also obtain nanocrystals in other shapes including polyhedrons and nanorod networks. The as-prepared pentacle nanocrystals can display strong LSPR peaks in the NIR region, which makes them possible potent agents for photothermal therapy. Upon irradiation by a NIR laser (808 nm, 1 W cm −2 ), the 70-nm pentacle nanocrystals exhibit a notable photothermal effect to kill 4T1 murine breast tumour cells. It is further discovered from photothermal treatment in vivo that 70-nm pentacle nanocrystals are able to regress the tumours on 4T1 tumour-bearing BALB/c mice. In addition, the pentacle Au–Cu alloy nanocrystals show better catalytic activity than polyhedrons and nanorod networks that are mostly enclosed by low-index facets towards the reduction of p -nitrophenol into p -aminophenol by sodium borohydride (NaBH 4 ). With sizes down to 70 and 45 nm, pentacle products appear to be even more active than conventional 5-nm Au nanoparticles. Our results show that pentacle Au–Cu alloy nanocrystals can be used as a versatile and diverse platform in biomedical applications owing to their tunable plasmonic properties, and that they have great potential as industrial catalysts. Structure and composition study The standard aqueous phase synthesis of pentacle Au–Cu alloy nanocrystals involves CuCl 2 and HAuCl 4 as precursors, glucose as the reductant and hexadecylamine (HDA) as the capping agent. At first, aqueous solutions of CuCl 2 , HAuCl 4 and glucose were added into a glass vial containing a mixture of HDA and deionized water. After being capped, the vial holding the final solution was magnetically stirred at room temperature overnight. It was then transferred into an oil bath and heated at 100 °C for 30 min. As the reaction proceeded, the solution changed its colour from kelly green to deep brown. 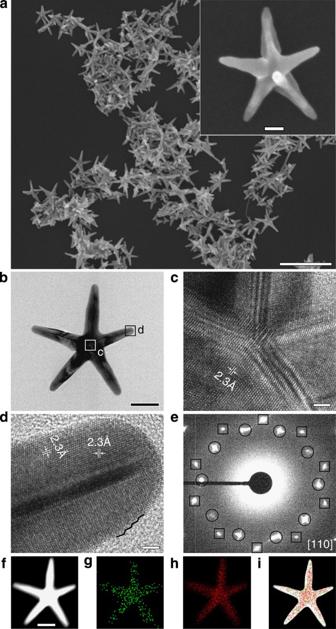Figure 1: Structure and composition study of pentacle Au–Cu alloy nanocrystals. (a) SEM image of the pentacle nanocrystals prepared through the standard procedure. The inset shows a SEM image of a typical individual nanocrystal. (b) TEM image of an individual pentacle Au–Cu alloy nanocrystal. (c,d) HRTEM images of the parts marked inb. (e) The corresponding selected-area electron diffraction pattern with the electron beam directed along the fivefold axis. The circles correspond to electron diffractions from the {111} planes while the boxes correspond to those from the {200} planes. (f) STEM image of a typical pentacle nanocrystal. (g,h) STEM-EDX elemental mapping image of (g) Cu and (h) Au of an individual pentacle Au–Cu alloy nanocrystal. (i) The merged image off,gandh. Scale bar, 500 nm (a) and 50 nm (b). Scale bar, 2 nm (c,d). Scale bar, 50 nm in the inset andf. Figure 1a shows a representative scanning electron microscopy (SEM) image of a sample prepared through the standard procedure, which indicates the purity and uniformity of the products. The nanocrystals consisted of five branches, which were 10–40 nm in width and 80–150 nm in length, with an angle of ~\n72° between adjacent ones. The inset, a magnified image to show a single particle, confirms the fivefold symmetric structure. To better substantiate, extra transmission electron microscopy (TEM) and SEM images of different individual pentacle nanocrystals are provided in Supplementary Fig. 1 . To visualize the crystalline structure of the as-prepared pentacle Au–Cu alloy nanocrystals, TEM and high-resolution TEM (HRTEM) analysis were conducted. Figure 1b shows a typical pentacle Au–Cu alloy nanocrystal on which HRTEM measurements were performed. Figure 1c,d shows HRTEM images recorded along the [110] zone axis, of the regions marked by boxes in Fig. 1b . In both images, periodic lattice fringes can be clearly seen. The lattice spacings marked around the core area ( Fig. 1c ) and branch ends ( Fig. 1d ) can all be indexed to {111} planes. As shown in Fig. 1d , the {111} twinning planes extended along to the end of the branch. Additional HRTEM images taken from different parts are integrated in Supplementary Fig. 2 to support an almost fivefold symmetric structure. Notably, the terraces on the edge marked with black lines in Fig. 1d probably correspond to high-index facets. Figure 1e shows the selected-area electron diffraction pattern obtained with the electron beam aligned parallel to the fivefold axis, that is, the [110] directions. It furnishes compelling evidence for the fivefold symmetric crystalline structure of the pentacle nanocrystals. The circles correspond to electron diffractions from the {111} planes while the boxes correspond to those from the {200} planes [38] . Figure 1f is a scanning TEM (STEM) image of a typical pentacle nanocrystal, on which elemental mapping analysis was induced. Figure 1g,h shows STEM-energy dispersive X-ray (STEM-EDX) elemental mapping of Cu and Au, respectively. The full coverage of both Cu and Au reveals the alloy structure. The merged image ( Fig. 1i ) further approves the complete overlapping of two metal components. The composition of pentacle nanocrystals was also examined by X-ray diffraction (XRD) and EDX spectra. As shown in Supplementary Fig. 3 , the XRD peaks of pentacle Au–Cu nanocrystals can be indexed as a face-centered cubic ( fcc ) structure, each of which lies in between that of pure fcc Au (JCPDS no. 04-0784) and pure fcc Cu (JCPDS no. 85-1326). Although XRD analysis backs the alloy structure, it remains difficult to deduce atomic content from it. Vegard’s law has been found unsuitable in the case of Cu and Au, because Cu may take the unusual interstitial position [28] . Supplementary Figure 4 shows the EDX spectrum, which confirms the elements of Au and Cu in the products (Mo came from the grids) and semi-quantitatively assesses the atomic percentage of Au and Cu to be 86.2% and 13.8%, respectively. Moreover, the atomic percentage of Au and Cu were determined to be 87.4% and 12.6% by inductive coupled plasma-atomic emission spectroscopy (ICP-AES), respectively. 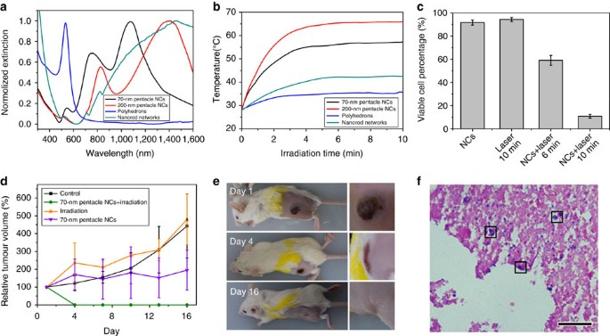Figure 4: Plasmonic properties of pentacle Au–Cu alloy nanocrystals and their applications in photothermal therapy. (a) Extinction spectra of aqueous suspensions of Au–Cu alloy nanocrystals with different shapes. (b) Photothermal effect of these Au–Cu alloy nanocrystals. The plot of temperature versus time was recorded upon irradiation by an 808-nm laser (1 W cm−2). (c) Viability of 4T1 murine breast tumour cells incubated under different conditions (with pentacle Au–Cu alloy nanocrystals or laser or both) for a specified period of time. The concentration of pentacle Au–Cu alloy nanocrystals was 10 μg ml−1, and the power density of the laser was 1 W cm−2. The incubation time of cells treated with only nanocrystals was 6 h. (d) The tumour growth curves of different groups of mice after treatment. The tumour volumes were normalized to their initial sizes. Laser wavelength=808 nm; power density=1 W cm−2; irradiation time=5 min. Error bars were based on s.d. of six mice per group. (e) Photographs of representative 4T1 tumour-bearing mice 1, 4 and 16 days after the photothermal treatment in the 70-nm pentacle nanocrystals+irradiation group. (f) Haematoxylin and eosin-stained tumour sections collected from a typical mice after 4-day photothermal treatment in the 70-nm pentacle nanocrystals+irradiation group. Characterized by loose structure and cells with pyknotic nuclei, necrosis was seen (black boxes inf). Scale bar, 20 μm (f). Figure 1: Structure and composition study of pentacle Au–Cu alloy nanocrystals. ( a ) SEM image of the pentacle nanocrystals prepared through the standard procedure. The inset shows a SEM image of a typical individual nanocrystal. ( b ) TEM image of an individual pentacle Au–Cu alloy nanocrystal. ( c , d ) HRTEM images of the parts marked in b . ( e ) The corresponding selected-area electron diffraction pattern with the electron beam directed along the fivefold axis. The circles correspond to electron diffractions from the {111} planes while the boxes correspond to those from the {200} planes. ( f ) STEM image of a typical pentacle nanocrystal. ( g , h ) STEM-EDX elemental mapping image of ( g ) Cu and ( h ) Au of an individual pentacle Au–Cu alloy nanocrystal. ( i ) The merged image of f , g and h . Scale bar, 500 nm ( a ) and 50 nm ( b ). Scale bar, 2 nm ( c , d ). Scale bar, 50 nm in the inset and f . Full size image Shape evolution Considering the rarely reported fivefold twinned structure of the as-prepared Au–Cu bimetallic nanocrystals, their nucleation and growth pathway is a valuable subject of research. Our investigation started from the TEM ( Supplementary Fig. 5 ) and HRTEM ( Fig. 2a,f ) images recorded from the samples prepared at different reaction time points. As shown in Fig. 2a ; Supplementary Fig. 5a , fivefold twinned seeds emerged at the initial stage of the reaction. The fivefold twinned nanocrystals on the length scale of several nanometers usually take three variants in shape, that is, the rounded decahedron, the Marks decahedron and the star decahedron [39] . According to this classification, the nanocrystals after reacting for 8 min are rounded decahedrons ( Fig. 2a ; Supplementary Fig. 5a ) and gradually grow into a novel type of larger decahedrons ( Fig. 2f ; Supplementary Fig. 5b ) that falls somewhere between the Marks decahedron and the star decahedron [39] , [40] . With the extension of reaction time to 20 ( Supplementary Fig. 5c ) and 30 min ( Supplementary Fig. 5d ), more and longer branches protruded from the twinning planes of the decahedral core, and the product became dominated by pentacle nanocrystals with an average branch length of 100 nm. The composition of these decahedral seeds was studied through STEM ( Fig. 2b,g ) aided by EDX mapping, which shows that both seeds at reaction time points of 8 and 12 min were alloys ( Fig. 2c,d,h,i ). As shown by line-scanning profiling analysis, both Cu and Au distributed nearly homogeneously across the decahedrons ( Fig. 2e,j ). 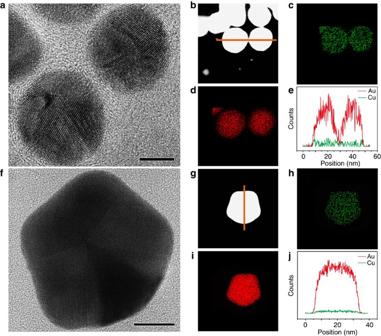Careful ICP-AES analysis ( Supplementary Table 1 ) shows that the atomic percentage of Cu rises from 4.7% (8 min) to 12.6% (30 min), upon which some rationale can be established for the formation of decahedral seeds and the following shape evolution. Figure 2: Characterization of decahedral seeds obtained at 8 and 12 min. (a,f) HRTEM images of rounded decahedrons obtained at 8 min and a decahedral seed obtained at 12 min. (b,g) STEM images of decahedral seeds obtained at 8 and 12 min, respectively. (c,d,h,i) STEM-EDX elemental mapping image of (c,h) Cu and (d,i) Au of decahedral seeds obtained at 8 and 12 min. (e,j) Elemental line-scanning profiles along the direction marked by orange lines inbandg, respectively. Scale bar, 10 nm (a) and 20 nm (f). Figure 2: Characterization of decahedral seeds obtained at 8 and 12 min. ( a , f ) HRTEM images of rounded decahedrons obtained at 8 min and a decahedral seed obtained at 12 min. ( b , g ) STEM images of decahedral seeds obtained at 8 and 12 min, respectively. ( c , d , h , i ) STEM-EDX elemental mapping image of ( c , h ) Cu and ( d , i ) Au of decahedral seeds obtained at 8 and 12 min. ( e , j ) Elemental line-scanning profiles along the direction marked by orange lines in b and g , respectively. Scale bar, 10 nm ( a ) and 20 nm ( f ). Full size image At the beginning of the reaction, metal precursors were quickly reduced by glucose. This especially applies to AuCl 4 − , because of the apparently higher redox potential of AuCl 4 − than Cu 2+ (Cu 2+ /Cu=0.342 V, AuCl 4 − /Au=1.002 V). The quick reaction gave rise to the formation of a large number of small seeds. It was pointed out by Yacamán et al. [39] that at nanometric sizes (typically ≤5 nm), the fivefold twinned structures such as icosahedrons and decahedrons tend to be more stable than cuboctahedrons [41] , [42] . Therefore, these seeds might take the shape of decahedrons as a result of thermodynamic preference. Owing to fast reduction, the amount of AuCl 4 − ions in the solution declined quickly, while that of Cu 2+ ions was still maintained at a relatively high level. Although the formation of decahedral seeds could be supported at the early stage, it became unsustainable at later time points. The growth mode was then dominated by kinetic control and deposition of reduced metal atoms was localized at more reactive sites to enlarge twinning planes, but not much on the facets. We hypothesize that, in our work, the exposed facets are more stable than twin boundaries because of underpotential deposition of Cu on Au seeds, similar to the report on controlling the shape of Au nanostructures via Ag + ions by Personick et al. [43] At this growth stage, the proportion that Cu 2+ ions contributed augmented over time, which is supported by the gradual increase of Cu content in the products. Because of the strong capping effect of amine residues on the apex ({110} facets on the top and the bottom) of decahedral seeds [40] , the growth along twining planes was more selective to the five edges to form pentacle structures, even at a cost of extra strain energy, rather than to the apex to form nanorods. An implication of the asynchronous reduction of two metal precursors is that the Au content might be higher inside than outside, which would give rise to an Au-rich core. However, we did not observe it ( Fig. 1f–i ) probably because of the diffusion of newly reduced (and reactive) Cu atoms from outward to inward. The diffusion of one metal into another is a plausible mechanism to reform the nanocrystals into alloys [29] . Formation mechanism To explore the mechanism involved in the formation of pentacle Au–Cu alloy nanocrystals, we devised a set of experiments using the standard procedure, except for the amount or type of the capping agent or reducing agent. Supplementary Fig. 6a,b shows that the products are highly sensitive to the amount of capping agent. With less HDA (30 mg), the products turned to be polyhedrons ( Supplementary Fig. 6a ). In contrast, as the amount of HDA was increased to 90 mg, the nanorod network ( Supplementary Fig. 6b ) evolved. While only a small amount of HDA is involved in the reaction, the addition of metal ions to the seeds will be faster, giving rise to nearly isotropic growth in all directions and eventually the formation of polyhedrons. On the contrary, with sufficient HDA, growth is restricted in many directions on the decahedral seeds except for the direction along the twinning plane, as a result of capping. Then the growth of branches overwhelms other places, leading to a nanorod network with unrestrained stretching of the branches [27] . Similar to the concentration of HDA, the amount of glucose (the reducing agent) was also found to play an important role in controlling the morphology of the Au–Cu alloy nanocrystals. As illustrated in Supplementary Fig. 7 , neither too much nor too little glucose could generate a suitable reduction rate to obtain pentacle nanocrystals in high purity. Besides, we investigated the effect of chain length of the capping agent on the final shape of products. As shown in Supplementary Fig. 6c , when dodecylamine served as the capping agent, irregular-shaped nanocrystals dominated the product. This is primarily because dodecylamine also has a reducing effect so that the nucleation process will occur at room temperature when the solution undergoes magnetic stirring overnight. The aforementioned analysis was further proved by the use of octadecylamine (ODA). As shown in Supplementary Fig. 6d , because of the similar capping effect of ODA with HDA, the pentacle structures appeared again when equal amount of ODA was added into the vial instead of HDA. For this bimetallic system, the Au/Cu molar ratio was confirmed to be a main factor in shaping the final products. Supplementary Figure 8 shows TEM images of the products obtained under the standard reaction condition, except that different Au/Cu molar ratios of precursors were used. The pentacle shape could only be preserved when the ratio is between 11:9 and 2:3 (the standard value is 1:1). However, the percentage of Cu could still be tuned from 4.0 to 17.5% ( Supplementary Fig. 8d,e ) as the molar ratio is changed from 11:9 to 2:3, indicating that the growth mode of pentacle products is rather accommodating. None of the other experiments could yield well-defined pentacle nanocrystals. Specifically, pure Au and pure Cu precursors led to the formation of sphere-like Au particles and cube-like Cu particles, respectively. Other intermediate molar ratios (3:1, 3:2, 11:9, 2:3, 1:2 and 1:5), however, either gave rise to broken pentacle nanocrystals (resembling multipods), dendritic nanocrystals or a mixture of various shapes. It is believed that Au/Cu molar ratio of precursors is strongly related to both the nucleation and growth kinetics, and therefore the final morphology of products. Size control Beyond the standard synthesis, we realized size control of the products, especially those with smaller dimensions. In the practice, we held the strategy of shortening the reaction time and inducing additional HDA (see Methods for detailed procedures). The drop in reaction time can cut the size of decahedral seeds. 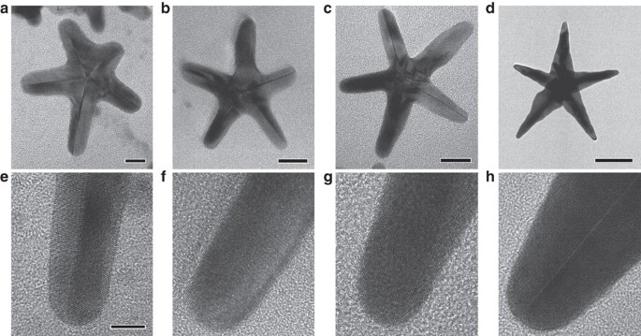The injection of HDA, in essence, can slow down the reaction rate after the formation of seeds, and therefore increase the selective growth of branches. Figure 3: TEM and HRTEM images of pentacle Au–Cu bimetallic nanocrystals with different sizes. (a–d) TEM images of individual pentacle Au–Cu alloy nanocrystals with sizes of 45, 70, 100 and 200 nm, respectively. (e–h) HRTEM images of the corresponding branches ina–d. Scale bar, 10, 20, 20 and 50 nm (a–d), respectively. Scale bar, 5 nm (e), which is also used forf,gandh. Figure 3a–d shows typical TEM images of individual pentacle Au–Cu bimetallic nanocrystals with sizes of ~\n45, 70, 100 and 200 nm, respectively. The four HRTEM images ( Fig. 3e–h ) show the corresponding branch ends of the products with different sizes. The width of branches generally increases with the overall size, while the fivefold twinned structure is largely preserved. The high-index feature is found to be definite, and stepped edges can be even more clearly identified owing to shorter branches than the standard products, as shown by higher magnification HRTEM images of the 45-nm and 100-nm products ( Supplementary Fig. 9 ). We have partially assigned the exposed high-index facets and found multiple sets of indices. The 45-nm product was chosen for EDX mapping analysis and the alloy structure was still confirmed ( Supplementary Fig. 10a–d ). Line-scanning profiles along different directions show that Cu and Au were uniformly distributed ( Supplementary Fig. 10e,f ). Figure 3: TEM and HRTEM images of pentacle Au–Cu bimetallic nanocrystals with different sizes. ( a – d ) TEM images of individual pentacle Au–Cu alloy nanocrystals with sizes of 45, 70, 100 and 200 nm, respectively. ( e – h ) HRTEM images of the corresponding branches in a – d . Scale bar, 10, 20, 20 and 50 nm ( a – d ), respectively. Scale bar, 5 nm ( e ), which is also used for f , g and h . Full size image Plasmonic properties and photothermal therapy (PTT) Motivated by the peculiar shapes and interesting surface properties, we investigated LSPR features of the as-prepared nanocrystals. Figure 4a is a combined graph of normalized extinction spectra of the as-prepared 70-nm and 200-nm pentacle nanocrystals, polyhedrons and nanorod networks in the range of 300–1,600 nm. For 70-nm pentacle nanocrystals, the strong peak at around 1,100 nm, the weaker peak at around 740 nm and the weak shoulder at around 550 nm, are likely attributed to dipole and high-order modes of LSPR, respectively. The corresponding peaks for 200-nm pentacle products were located at 1,400, 810 and 530 nm, respectively. The well-defined absorption peak in the NIR region inspired us to study the photothermal effect of the as-prepared nanocrystals. The photothermal effect was examined through measuring the temperature of 250 μl aqueous solutions of different types of nanocrystals with the same concentration (10 μg ml −1 ), irradiated by a NIR laser (808 nm, 1 W cm −2 ) over time. As shown in Fig. 4b , the temperature of the solution containing 70-nm pentacle nanocrystals rose from 28 to 55 °C within 10 min, the increase of which greatly exceeds the two counterparts of polyhedrons and nanorod networks. The temperature rise in the solution of 200-nm pentacle nanocrystals was slightly higher than that of 70-nm nanocrystals, partly because the NIR peak for 200-nm nanocrystals was more matching with the wavelength of the laser. Figure 4: Plasmonic properties of pentacle Au–Cu alloy nanocrystals and their applications in photothermal therapy. ( a ) Extinction spectra of aqueous suspensions of Au–Cu alloy nanocrystals with different shapes. ( b ) Photothermal effect of these Au–Cu alloy nanocrystals. The plot of temperature versus time was recorded upon irradiation by an 808-nm laser (1 W cm −2 ). ( c ) Viability of 4T1 murine breast tumour cells incubated under different conditions (with pentacle Au–Cu alloy nanocrystals or laser or both) for a specified period of time. The concentration of pentacle Au–Cu alloy nanocrystals was 10 μg ml −1 , and the power density of the laser was 1 W cm −2 . The incubation time of cells treated with only nanocrystals was 6 h. ( d ) The tumour growth curves of different groups of mice after treatment. The tumour volumes were normalized to their initial sizes. Laser wavelength=808 nm; power density=1 W cm −2 ; irradiation time=5 min. Error bars were based on s.d. of six mice per group. ( e ) Photographs of representative 4T1 tumour-bearing mice 1, 4 and 16 days after the photothermal treatment in the 70-nm pentacle nanocrystals+irradiation group. ( f ) Haematoxylin and eosin-stained tumour sections collected from a typical mice after 4-day photothermal treatment in the 70-nm pentacle nanocrystals+irradiation group. Characterized by loose structure and cells with pyknotic nuclei, necrosis was seen (black boxes in f ). Scale bar, 20 μm ( f ). Full size image Despite that, 70-nm pentacle nanocrystals showed a slightly weaker photothermal effect than 200-nm products, their smaller size are likely to circumvent reticuloendothelial system (RES) uptake, making them more appropriate for tumoricidal applications [44] . We initially tested the ability of 70-nm pentacle nanocrystals for photothermal treatment of 4T1 murine breast tumour cells in vitro . The photothermal efficiency of killing cancer cells was measured by standard 3-(4,5-dimethylthiazol-2-yl)-2,5-diphenyltetrazolium bromide (MTT) assay. As shown in the bar chart of viability ( Fig. 4c ), after incubation with 70-nm pentacle nanocrystals and without irradiation for 6 h, >90% of the 4T1 cells survived. In another experiment, the viable percentage of 4T1 cells without adding nanocrystals remained ~\n95% after 10 min of exposure to irradiation by the 808-nm laser (power density=1 W cm −2 ). By comparison, the exposure of 4T1 cells to 10 μg ml −1 of pentacle nanocrystals with the presence of irradiation led to a quick decline in viability. Supplementary Fig. 11a–c shows micrographs of the 4T1 cells after 0, 6 and 10 min of irradiation, respectively. The dead cells are stained with propidium iodide. It was found that >40% of the cells were killed after 6 min of irradiation and nearly 90% were killed after 10 min of laser treatment ( Fig. 4c ). For in vivo PTT study, we employed subcutaneous 4T1 xenograft model in BALB/c mice to study the efficacy of photothermal treatment of 70-nm pentacle nanocrystals. Twenty-four tumour mice were randomly and evenly divided into four groups, which were the control group with no particular treatment, the group with intratumoral injection of 70-nm pentacle nanocrystals and irradiation of NIR laser (808 nm, 1 W cm −2 ) for 5 min, the group with only irradiation and the group with only particle injection. Supplementary Figure 12 shows infrared radiation thermal images of tumour-bearing BALB/c mice at different time points of irradiation, which confirms the in vivo photothermal effect. Supplementary Figure 13 shows photographs of mice and their close-up views of tumours in four differently treated groups at day 4, with one representative mouse from each group. It is clearly observed that the thorough regression of tumour was only found in the photothermal group. Figure 4d compares the change in relative tumour volume (that is, normalized against initial values before treatment) on BALB/c mice along with feeding time. In the control experiment, the tumours grew exponentially to >3 times larger in 2 weeks than those in 1 day. As shown by red and purple segmental lines, the tumours from both the irradiation-only and injection-only groups enlarged in volume, with some fluctuations. These experiments ruled out the possibility that any single factor can effectively suppress tumour growth. The group of mice that received both nanocrystal injection and irradiation, however, was rid of tumours 4 days after the treatment ( Fig. 4e ; Supplementary Fig. 13 ). To understand the effect of PTT at a microscopic perspective, we studied the existence of cancer cells in the tumours of differently treated mice by tissue slicing and staining. Since well-differentiated glandular cancer cells are characterized by a large cell nucleus, which is one to five times larger than those of the normal cells and abundant cytoplasm, it is not difficult to identify them under the optical microscope. In our experiments, densely distributed cancer cells could be found in tumour sections collected from non-photothermally treated mice ( Supplementary Fig. 14a–c ). They are with visibly big nuclei that are usually darker than the cytoplasm. Figure 4f , which is a partially enlarged view of Supplementary Fig. 14d , however, shows separation of pyknotic nuclei from the cytoplasm (marked by black boxes). This result demonstrates necrosis of the tumour and thus the effectiveness of photothermal therapy to 4T1 tumour. We also examined the influence of injected metal nanocrystals on major organs of the mice. As shown in Supplementary Fig. 15 , no obvious abnormality was found from haematoxylin and eosin-stained images of the major organs of the as-treated mice at day 1, with those of the untreated mice as a benchmark. Encouraged by the high NIR absorbance and strong PTT efficacy of pentacle nanocrystals, we attempted delivering the 70-nm pentacle Au–Cu nanocrystals to tumours via systemic intravenous injection. The surface of pentacle nanocrystals was coated with a monolayer of polyethylene glycol (PEG), which allows a long circulation time of pentacle nanocrystals in the blood stream and accumulation in the tumour. Two groups of mice (three mice per group), which received either an intravenous injection of PEGylated nanocrystals (1 mg ml −1 , 200 μl) or saline (2 mg ml −1 , 20 μl), were compared for photothermal heating efficiency. At 1 day post injection, both groups of mice were irradiated by a NIR laser for 6 min and the temperature change in the tumour area under NIR irradiation was recorded. The tumour surface temperatures rapidly increased (up to 6.14±0.86 °C) in the group treated with PEGylated nanocrystals, but the control group showed little change ( Supplementary Fig. 16 ). The passive tumour accumulation of PEGylated nanocrystals after intravenous injection could be attributed to the enhanced permeability and retention effect of tumours [45] , indicating the tumour diagnostic and therapeutic potential of pentacle nanocrystals. Catalytic properties Owing to the synergistic effect of the two metal components, large surface area of the branches and possibly high-index facets, the pentacle Au–Cu alloy nanocrystals are expected to exhibit excellent catalytic effect towards a wide range of reactions [30] , [33] . We adopted the reduction of p -nitrophenol to p -aminophenol by NaBH 4 as a model reaction to evaluate the catalytic activity of differently sized products [46] , [47] , [48] . To set points of reference, polyhedrons ( Supplementary Fig. 6a ), nanorod network ( Supplementary Fig. 6b ) and conventional citrate-coated Au nanoparticles ( Supplementary Fig. 17 ) were tested under the same conditions. The well-established reaction has been reported to be catalysed by a variety of noble metal nanocrystals and the reaction kinetics can be monitored by spectroscopic measurements. 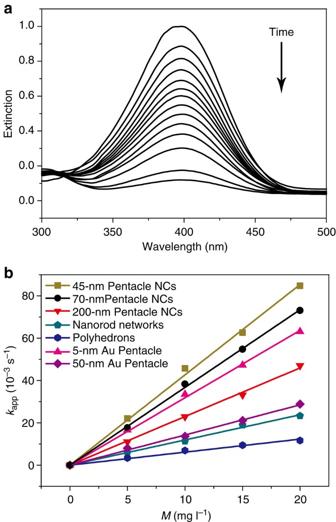Figure 5: Catalytic properties of pentacle Au–Cu alloy nanocrystals. (a) The extinction spectra recorded at different reaction time points, indicating the disappearance of the peak forp-nitrophenol owing to the reduction of -NO2group into -NH2group. (b) Plots of the apparent rate constants (kapp) as a function of the mass concentration (M), relating to the use of different types of Au–Cu bimetallic nanocrystals and conventional Au nanoparticles as catalysts for the reduction ofp-nitrophenol intop-aminophenol by NaBH4. Figure 5a shows a typical set of extinction spectra recorded at different time points of the reaction, which has been normalized against the extinction intensity before the reaction. Under a neutral or acidic condition, p -nitrophenol solution should exhibit a strong absorption peak at 317 nm. With the addition of NaBH 4 , p -nitrophenolate ions will take the lead as the alkalinity of the solution increases and then the absorption peak redshifts to ~\n400 nm (ref. 49 ). This analysis explains the peak position at the initial time point. After the addition of catalysts, a new peak at 315 nm for p -aminophenol appeared, and the intensity of the absorption peak at 400 nm gradually lowered as increasing amount of p -nitrophenol was reduced to p -aminophenol. Because the peak at 400 nm dominated for most of the time, it is reasonable to derive the concentration of p -nitrophenolate ions from absorbance at 400 nm and thus to investigate the reaction kinetics. It should be noted that all experiments were accomplished with fixed concentrations of p -nitrophenol (1.4 × 10 −4 M) and NaBH 4 (4.2 × 10 −2 M). Because the concentration of NaBH 4 is comparatively enormous compared with p -nitrophenol, it is considered as a constant during the reaction. Therein, we assume that the pseudo-first-order kinetics with respect to p -nitrophenol (or p -nitrophenolate) can be applied, which is supported by the linear relationship between the logarithm of the normalized extinction intensity at 400 nm and time (minus adsorption time). Therefore, we are able to calculate the apparent reaction rate constants ( k app ) in reaction systems with different concentrations and types of metal nanocrystals using the previously reported method [47] , [48] . The apparent rate constant versus mass concentration ( M ) appears in a linear relationship ( Fig. 5b ). To exclude the influence of volume change and thus different concentrations of nanocrystals, we further derived the slope of the line ( k 1 ) from the equation of first-order kinetics (see equation (1)), which reflects the intrinsic catalytic activity. Figure 5: Catalytic properties of pentacle Au–Cu alloy nanocrystals. ( a ) The extinction spectra recorded at different reaction time points, indicating the disappearance of the peak for p -nitrophenol owing to the reduction of -NO 2 group into -NH 2 group. ( b ) Plots of the apparent rate constants ( k app ) as a function of the mass concentration ( M ), relating to the use of different types of Au–Cu bimetallic nanocrystals and conventional Au nanoparticles as catalysts for the reduction of p -nitrophenol into p -aminophenol by NaBH 4 . Full size image The slope ( k 1 ) related to 200-nm pentacle nanocrystals, nanorod networks and polyhedrons were determined to be 2.30 × 10 −3 , 1.19 × 10 −3 and 0.61 × 10 −3 l s −1 mg −1 , respectively. Therefore, 200-nm pentacle nanocrystals enjoyed higher level of catalytic activity than Au–Cu bimetallic nanocrystals in the other two shapes. As shown in Fig. 5b , although conventional Au nanoparticles appeared less active than 200-nm pentacle nanocrystals at a size of 50 nm, they gave substantially higher activity with a smaller dimension (5 nm in size), which was higher than what the 200-nm pentacle nanocrystals could offer. The comparative study on size dependence of catalytic activities of pentacle nanocrystals shows that k 1 climbed up from 2.30 × 10 −3 to 3.67 × 10 −3 and 4.27 × 10 −3 l s −1 mg −1 , respectively, as the size was reduced to 70 and 45 nm. Obviously, the activities of 70-nm and 45-nm pentacle nanocrystals were both higher than 5-nm conventional Au nanoparticles. It can thus be concluded that the advantages brought about by the synergistic effect, twinning interfaces and possibly the high-index feature could overcome significantly smaller surface area/volume ratio. We further addressed the relationship between apparent reaction rate and surface area concentration to discern specific activities with respect to surface area. The surface areas of different types of Au–Cu bimetallic nanocrystals were calculated on schematic models ( Supplementary Fig. 18 ). It was interesting to find that the specific activity per area of pentacle nanocrystals dropped with size ( Supplementary Fig. 19 ). An intuitive explanation may be that, larger pentacle nanocrystals had a bigger portion of exposed high-index facets on branches, which might serve as highly active sites for catalysis. However, the specific reaction rate constant with regard to 45-nm pentacle nanocrystals was still higher than those of the other two kinds of Au–Cu bimetallic nanocrystals. This may illustrate that a small proportion of exposed high-index facets could promote total activity towards the reaction. In summary, we report a facile aqueous synthetic route to pentacle Au–Cu alloy nanocrystals with fivefold twinning. Through manipulating the reaction time and the addition of capping agent, we obtained pentacle-shaped products with tunable size from 45 to 200 nm. According to electron microscopic analysis of the samples obtained at different reaction time points, decahedral seeds formed at the initial stage of the reaction, and then multiple branches protruded parallel to the twinning planes. Study on the formation mechanism revealed that unduly large or small amounts of capping agent or reducing agent might prevent the formation of well-defined pentacle nanocrystals and create other shapes, including polyhedrons and nanorod networks. The as-prepared pentacle nanocrystals displayed strong LSPR properties in the NIR region, which created an obvious photothermal effect. It was demonstrated that upon NIR irradiation, 4T1 murine breast tumour cells incubated with 70-nm pentacle nanocrystals were effectively killed. Further in vivo study showed the photothermal destruction of 4T1 murine breast tumour grown on BALB/c mice. In catalysis tests, pentacle nanocrystals exhibited higher catalytic activity than polyhedrons and nanorod networks towards a model reaction of reducing p -nitrophenol by NaBH 4 . Although they appeared less competitive in activity than 5-nm conventional citrate-coated Au nanoparticles at the size of 200 nm, pentacle nanocrystals were more active than 5-nm conventional Au nanoparticles with reduced sizes to 70 and 45 nm. We believe this piece of work can provide an insight into the aqueous phase synthesis of bimetallic nanocrystals and promote their applications in biomedicine and catalysis. Chemicals and materials Cupric chloride dihydrate (CuCl 2 ·2H 2 O, 99%), tetrachloroaurate trihydrate (HAuCl 4 ·3H 2 O, 99%) and glucose (α or β form) were purchased from Sinopharm Chemical Reagent Co. Ltd (Shanghai, China). HDA (90%) was obtained from Sigma-Aldrich. All the vials were made from borosilicate glass, with a black phenolic-moulded screw cap and polyvinyl-faced pulp liner. Ultrapure Millipore water (18.2 MΩ) was used as the solvent throughout. Synthesis of 200-nm pentacle Au–Cu alloy nanocrystals In a standard synthesis of pentacle Au–Cu alloy nanocrystals, 0.3 ml of aqueous CuCl 2 ·2H 2 O (100 mM), 0.3 ml of aqueous HAuCl 4 ·3H 2 O (100 mM), 45 mg of HDA, 0.28 ml of aqueous glucose (1 M) and 4 ml of water were added in a 20-ml vial at room temperature. After the vial had been capped, the solution was magnetically stirred at room temperature overnight. The capped vial was then transferred into an oil bath and heated at 100 °C for 30 min under magnetic stirring. As the reaction proceeded, the solution changed its colour from kelly green to brown. To prepare samples for electron microscopy characterizations, the pentacle nanocrystals were centrifugated at 10,000 r.p.m. for 8 min and washed with water three times and ethanol twice to remove excess precursor, HDA and glucose. As discussed in the main text, the shapes of the Au–Cu nanocrystals could be controlled to polyhedrons and nanorod networks by simply adjusting the concentrations of HDA. Controlling the size of pentacle Au–Cu alloy nanocrystals In a synthesis of 45-nm pentacle Au–Cu alloy nanocrystals, 0.3 ml of aqueous CuCl 2 ·2H 2 O (100 mM), 0.3 ml of aqueous HAuCl 4 ·3H 2 O (100 mM), 45 mg of HDA, 0.28 ml of aqueous glucose (1 M) and 4 ml of water were added in a 20-ml vial at room temperature. After the vial had been capped, the solution was magnetically stirred at room temperature overnight. The capped vial was then transferred into an oil bath and heated at 100 °C for 3 min. Then 30 mg HDA was added into the reaction solution at 100 °C. The reaction was stopped and the solution was cooled down using iced water when its colour changed from kelly green to brown. The 70-nm and 100-nm pentacle Au–Cu alloy nanocrystals were prepared under the same condition with 45-nm ones, except for the heating time before the addition of HDA extended to 4 and 5 min, respectively. Characterizations SEM images were obtained with a SEM (JSM-6700F) operated at 5 kV. TEM and HRTEM images were collected on a JEOL ARM-200F field-emission transmission electron microscope operating at 200 kV accelerating voltage. XRD characterization was performed using a Philips X'Pert Pro X-ray diffractometer with a monochromatized Cu Kα radiation source and a wavelength of 0.1542, nm. ICP-AES (Atomscan Advantage, Thermo Jarrell Ash, USA) was used to determine the concentration of Au and Cu. Extinction spectra were recorded on a U-4100 at room temperature (Hitachi, Japan). Photothermal effect measurement To study the photothermal effect induced by the NIR laser, 250-μl solutions containing 10 μg ml −1 Au–Cu alloy nanocrystals with three different sizes or shapes were irradiated by a NIR laser (808 nm, 1 W cm −2 ). The temperatures of the solutions were monitored by a thermocouple microprobe ( ϕ =0.5 mm) submerged in the solution in a hole of a 96-well plate. The probe was placed at such a position that the direct irradiation of the laser on the probe was avoided. Apoptosis assay 4T1 cells were cultured in RPMI 1640 medium in 96-well plates. The cell density was 1 × 10 5 cells per well. After being seeded for 18 h, the media were replaced by culture media containing 10 μg ml −1 pentacle Au–Cu alloy nanocrystals. The incubations were carried out at 37 °C in 5% CO 2 atmosphere for 6 h. After incubation, cell viabilities were measured by the standard MTT assay, a colorimetric assay based on the ability of viable cells to reduce 3-[4,5-dimethylthiazol-2-yl]-2,5-diphenyltetrazolium bromide. The survival rate and the error bar are shown in Fig. 4c (the case of incubating with nanocrystals only). Photothermal killing of cancer cells After incubation with 10 μg ml −1 pentacle Au–Cu alloy nanocrystals, 4T1 cells were exposed to a 1-W cm −2 808-nm laser for various periods to induce photothermal cell damage. For comparison, we also put the 4T1 cells under the same laser condition for 10 min. To identify the cell viability, the dead cells were stained with propidium iodide ( Supplementary Fig. 11 ). Cell viabilities were also measured by the standard MTT assay. Animal model BALB/c mice (~\n20 g ) were used under protocols approved by the Xiamen University Laboratory Animal Center. For the 4T1 murine breast tumour model, about 5 × 10 6 4T1 cells in 60 μl of phosphate-buffered saline were injected subcutaneously into the flank of the mouse. The mice were used when their tumour volumes reached 60–70 mm 3 . In vivo photothermal therapy An optical fibre-coupled 808-nm high power diode-laser was used to irradiate tumours during experiments. For photothermal treatment, BALB/c mice bearing 4T1 murine breast tumours were intratumorally injected with Au–Cu alloy nanocrystals (30 μl of 1 mg ml −1 solution for each mouse) at the power density of 1 W cm −2 for 5 min. Infrared thermal images were taken by an ICI 7320 Pro thermal imaging camera. The tumour sizes were measured by a caliper every other day and calculated as volume=(tumour length) × (tumour width) 2 /2. Relative tumour volumes were calculated as V / V 0 ( V 0 is the tumour volume when the treatment was initiated). Tissue slicing and staining To obtain tissue sections, three mice from each group were killed at different days. Tumours or major organs from these mice were fixed in 10% neutral-buffered formalin, processed routinely into paraffin, sectioned at 5 μm, stained with haematoxylin and eosin and then examined by a digital microscope. For Fig. 4f ; Supplementary Fig. 14 , tumours were collected at day 4. For Supplementary Fig. 15 , tissues were obtained at day 1, from heart, liver, kidney, lung, spleen stomach and pancreas. In vivo thermographic profiling Mice bearing 4T1 tumours 1 day post intravenous injection with 200 μl of 1 mg ml −1 PEGylated pentacle Au–Cu alloy nanocrystals or saline were anaesthetised and exposed to be irradiated by a NIR laser (808 nm, 1 W cm −2 ) for 6 min. During irradiation, the tumour surface temperatures were recorded by an infrared radiation thermal camera. Testing of catalytic properties For all experiments, the initial concentrations of p -nitrophenol and NaBH 4 were kept at 1.4 × 10 −4 and 4.2 × 10 −2 M, respectively. The mass concentrations of Au–Cu alloy catalysts were calculated depending on ICP-AES measurement. For polyhedrons and nanorod networks, the atomic percentages of Cu/Au were 10.1%/89.9% and 11.5%/88.5%, respectively. For pentacle nanocrystals, the result is provided in the main text. For accuracy, the extinction caused by the Au nanoparticles and the Au–Cu alloy catalysts was subtracted from all the spectroscopic measurements. How to cite this article: He, R. et al. Facile synthesis of pentacle gold–copper alloy nanocrystals and their plasmonic and catalytic properties. Nat. Commun. 5:4327 doi: 10.1038/ncomms5327 (2014).